Unidirectional transfer of microRNA-loaded exosomes from T cells to antigen-presenting cells The immune synapse is an exquisitely evolved means of communication between T cells and antigen-presenting cells (APCs) during antigen recognition. Recent evidence points to the transfer of RNA via exosomes as a novel mode of intercellular communication. Here we show that exosomes of T, B and dendritic immune cells contain microRNA (miRNA) repertoires that differ from those of their parent cells. We investigate whether miRNAs are exchanged during cognate immune interactions, and demonstrate the existence of antigen-driven unidirectional transfer of miRNAs from the T cell to the APC, mediated by the delivery of CD63+ exosomes on immune synapse formation. Inhibition of exosome production by targeting neutral sphingomyelinase-2 impairs transfer of miRNAs to APCs. Moreover, miRNAs transferred during immune synapsis are able to modulate gene expression in recipient cells. Thus, our results support a mechanism of cellular communication involving antigen-dependent, unidirectional intercellular transfer of miRNAs by exosomes during immune synapsis. To mount an effective immune response, different immune cell types need to communicate with each other. Cell synapses are highly specific means of intercellular communication. During the formation of the immunological synapse (IS), transmembrane and membrane-associated molecules are reorganized into a highly segregated structure at the T cell–antigen-presenting cell (APC) contact site [1] , [2] . The actin cytoskeleton reorganizes to provide a physical platform to support the IS structure, whereas the tubulin cytoskeleton is directed towards the IS, where the microtubule-organizing centre (MTOC) localizes [3] , [4] . The translocation of the MTOC is an early event during IS formation, and allows localization of the secretory compartments—the Golgi apparatus and the cytotoxic granules—in close apposition to the APC. The polarization of the secretory apparatus to the IS provides the basis for polarized secretion of cytokines [3] , [5] and the exocytosis of lytic granules by cytotoxic T cells [6] . An alternative vesicular trafficking, depending on the endocytic pathway, has also been reported to be critical for IS function. Transport of the T cell receptor (TCR) [7] and lymphocyte-specific tyrosine kinase [8] to the IS depends on components of the endosomal compartments, and endosomal transport is essential both to target TCRs and other molecules to the APC contact site and for signal downmodulation by controlling TCR endocytosis. Finally, lysobisphosphatidic acid, a marker of late endosomes (multivesicular bodies; MVBs), localizes very close to the centre of the IS of helper T cells [9] , suggesting that MVBs also polarize to the IS. The IS may thus serve as a focus for both exocytosis and endocytosis [6] , [10] . On exocytic fusion of MVBs with the plasma membrane, cells release exosomes; and these 30–100 nm vesicles are increasingly recognized as significant vehicles for intercellular communication [11] , [12] . The generation of MVBs is a well-defined event in the endosomal pathway and it is evident that they have a dual role, as in addition to their involvement in exosomal release MVBs also temporarily store proteins and lipids destined for lysosomal degradation [11] . The role of exosomes in diverse physiological and pathological settings is still incompletely understood; however, evidence has been reported for their involvement in important processes, such as antigen presentation, tumour immunity and the transmission of infectious agents [12] . Exosomes contain a characteristic composition of proteins, and express cell recognition molecules on their surface that facilitate their selective targeting of and uptake by recipient cells. Recent reports indicate that exosomes also harbour a variety of mRNAs and microRNAs (miRNA) [13] , [14] , which can be transferred to recipient cells and modulate their function [13] , [14] , [15] , [16] , [17] , [18] . These findings have increased interest in the role of exosomes in cell-to-cell communication, and support the idea that exosomes might constitute an exquisite mechanism for local and systemic intercellular transfer not only of proteins but also of genetic information in the form of RNA [11] , [12] , [19] . MiRNAs are a large family of small (22–24 nucleotides long), non-coding RNAs that downregulate gene expression by preventing the translation of specific mRNA into protein [20] . The emergence of miRNAs as potent post-transcriptional regulators of gene expression has broad implications in all areas of cell biology, including the immune system [21] , [22] , [23] . For example, specific miRNAs such as miR-155 and miR-181 regulate both the immune response and immune system development [24] , [25] , [26] . In addition, genetic ablation of the whole miRNA machinery or specific miRNAs severely compromises immune development and can lead to autoimmune disorders and cancer [27] , [28] . Here we present evidence that exosomes mediate antigen-driven unidirectional transfer of miRNAs from the T cell to the APC during T cell–APC cognate immune interactions. Moreover, our data indicate that miRNAs transferred on immune synapsis can be functional in the recipient cell. MiRNA profiles of immune cells and their exosomes To determine the miRNA repertoires of exosomes secreted by immune cells, we isolated exosomes from cell supernatants of the Raji B-cell line, the Jurkat-derived J77 T cell line, and primary dendritic cells (DCs) derived from human monocytes. Exosomes were isolated by a series of microfiltration and ultracentrifugation steps [29] , and exosome identity was assessed by extensive protein analysis with liquid chromatography with tandem mass spectrometry (LC MS/MS) technology. About 60% of proteins found in the analysed exosome samples have been previously found in other types of exosomes; these include the tetraspanins CD63, CD81 and CD9, proteins involved in membrane transport and fusion (Rab GTPases, annexins and fotillin), and other exosomal markers such as Tsg101 (data not shown). Moreover, exosomes derived from T lymphocytes and from APCs both contained RNA. Profiling of RNA isolated from exosomes and their donor cells indicates that exosomes are highly enriched in small RNA species ( Supplementary Fig. S1 ). Agilent microRNA microarray analysis (Agilent) showed that certain miRNAs are expressed at higher levels in exosomes than in their donor cells and vice versa ( Fig. 1 and Supplementary Data 1 ). The hierarchical clustering and the principal component analysis of the array data grouped the samples according to their cellular or exosomal origin ( Fig. 1a,b ). Several miRNAs (for example, miR-760, miR-632, miR-654-5p and miR-671-5p) were significantly more abundant in exosomal samples from all cell types; others, for example miR-335, were found only in exosomes derived from the primary DCs; in contrast, others (for example, miR-101, miR-32 and miR-21*) were more highly represented in cells than in exosomes ( Fig. 1c ). These data indicate that specific miRNA populations are selectively sorted into exosomes. Consistently, there was lower overall similarity between the miRNA repertoire in exosomes and their corresponding cells than between the exosomes of different cellular origin ( Fig. 1d ). 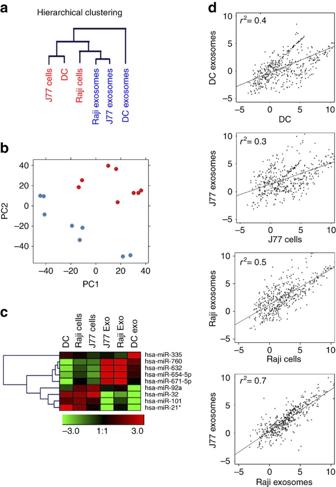Figure 1: microRNA profiles of exosomes and their parental cells. (a) Microarray analysis of exosomal miRNAs versus the miRNAs of their respective donor cells. Exosomes were isolated by serial centrifugation and filtration steps from supernatants of donor cells cultured in RPMI-1640 supplemented with exosome-depleted FBS (10%). Total RNA, including microRNA, was isolated from exosomes and their donor cells and miRNA profiles were assessed by microarray technology. The panel shows the hierarchical clustering of the VSN-normalized array data in the log2 scale averaged per biological replicate for each origin (exosomes per cells) and cell type. DC, dendritic cells; J77, Jurkat-derived J77 T cell line; Raji, Raji B cell line). (b) Principal component analysis (PCA) of all normalized array data. Each point represents a hybridized sample: that is, different biological samples per origin and cell type.xaxis, first principal component (PC1);yaxis, second principal component (PC2). Cell samples, red; exosomal samples, blue. (c) Heatmap of the VSN-normalized data for selected miRNAs. For visualization purposes the expression profiles were centred on the median of the profile. The scale bar across the bottom depicts standard deviation change from the mean. (d) Scatter plots of the exosome versus cell averaged array data in each cell type and of Raji exosomes versus J77 exosomes. The correlation is shown. Figure 1: microRNA profiles of exosomes and their parental cells. ( a ) Microarray analysis of exosomal miRNAs versus the miRNAs of their respective donor cells. Exosomes were isolated by serial centrifugation and filtration steps from supernatants of donor cells cultured in RPMI-1640 supplemented with exosome-depleted FBS (10%). Total RNA, including microRNA, was isolated from exosomes and their donor cells and miRNA profiles were assessed by microarray technology. The panel shows the hierarchical clustering of the VSN-normalized array data in the log2 scale averaged per biological replicate for each origin (exosomes per cells) and cell type. DC, dendritic cells; J77, Jurkat-derived J77 T cell line; Raji, Raji B cell line). ( b ) Principal component analysis (PCA) of all normalized array data. Each point represents a hybridized sample: that is, different biological samples per origin and cell type. x axis, first principal component (PC1); y axis, second principal component (PC2). Cell samples, red; exosomal samples, blue. ( c ) Heatmap of the VSN-normalized data for selected miRNAs. For visualization purposes the expression profiles were centred on the median of the profile. The scale bar across the bottom depicts standard deviation change from the mean. ( d ) Scatter plots of the exosome versus cell averaged array data in each cell type and of Raji exosomes versus J77 exosomes. The correlation is shown. Full size image Multivesicular bodies from T lymphocytes polarize towards the IS To analyse the capacity of cells to take up immune exosomes, we generated Raji B and J77 T cells stably expressing the exosomal marker CD63 fused to green fluorescent protein (GFP). The tetraspanin CD63 is very abundant in exosomes, and inside cells localizes mainly to MVBs and lysosomes, with only a small pool present at the plasma membrane [30] . Cytometry and western blot analyses confirmed the presence of CD63-GFP in exosomes released by these cells ( Fig. 2a and Supplementary Fig. S2 ). The purified CD63-GFP exosomes were then incubated with non-transfected J77 cells or Raji cells (recipient cells) for 16 h. Flow cytometry analysis revealed that both J77 T and Raji B cells have the capacity to take up immune exosomes ( Fig. 2b ). It is important to highlight that Raji B cells take up T cell-derived exosomes to a greater extent than their own exosomes and vice versa . Moreover, CD63-GFP was detected at the surface of recipient cells by confocal microscopy ( Fig. 2c ), suggesting that exosomes are not internalized but remain attached to the recipient plasma membrane. 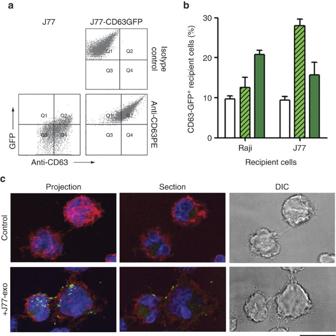Figure 2: Uptake of CD63-GFP exosomes by immune cells. (a) Untransfected J77 T cells and J77 T cells stably expressing CD63-GFP (J77-CD63-GFP cells) were cultured in exosome-depleted medium for 24 h and exosomes were purified from supernatants by ultracentrifugation. Exosomes were labelled with anti-CD63-phycoerythrin and analysed by flow cytometry. (b) Uptake of CD63-GFP exosomes by T cells and B cells (recipient cells). Untransfected cells were incubated with CD63-GFP exosomes for 16 h and analysed by flow cytometry. Data represent the percentage of GFP-positive cells (±s.e.m.) of three independent experiments. Open bars, no exosomes; striped bars, Raji exosomes; filled bars, J77 exosomes. (c) Confocal microscopy detection of CD63-GFP (green) on the surface of recipient cells (Raji) after incubation with J77-CD63-GFP exosomes. Cell membranes were stained for the cell-surface molecule CD45 (red) and nuclei were stained with HOESCHT (blue). Images show maximal projections of confocal images (projection), one representative confocal section (section) and the DIC images. Scale bar, 10 ìm. Figure 2: Uptake of CD63-GFP exosomes by immune cells. ( a ) Untransfected J77 T cells and J77 T cells stably expressing CD63-GFP (J77-CD63-GFP cells) were cultured in exosome-depleted medium for 24 h and exosomes were purified from supernatants by ultracentrifugation. Exosomes were labelled with anti-CD63-phycoerythrin and analysed by flow cytometry. ( b ) Uptake of CD63-GFP exosomes by T cells and B cells (recipient cells). Untransfected cells were incubated with CD63-GFP exosomes for 16 h and analysed by flow cytometry. Data represent the percentage of GFP-positive cells (±s.e.m.) of three independent experiments. Open bars, no exosomes; striped bars, Raji exosomes; filled bars, J77 exosomes. ( c ) Confocal microscopy detection of CD63-GFP (green) on the surface of recipient cells (Raji) after incubation with J77-CD63-GFP exosomes. Cell membranes were stained for the cell-surface molecule CD45 (red) and nuclei were stained with HOESCHT (blue). Images show maximal projections of confocal images (projection), one representative confocal section (section) and the DIC images. Scale bar, 10 ìm. Full size image To address whether exosomes mediate the transfer of miRNA during cognate immune interactions, we first studied the intracellular distribution of MVBs—the compartments from which exosomes arise—during the formation of an IS. In these experiments, Raji B cells were pulsed with Staphylococcus enterotoxin superantigen-E (SEE) and then incubated with TCR-Vβ8 + J77 T cells. MVB localization was assessed by immunofluorescence analysis of CD63 and two components of the ESCRT (endosomal sorting complex required for transport): Hrs, a component of the ESCRT-0 complex; and the late acting ESCRT machinery component VPS4. In the presence of SEE, which promotes formation of a fully functional IS, the MVBs of the J77 T lymphocyte lost their random cytoplasmic distribution and congregated near the IS (identified by CD3 and actin staining); in contrast, the localization of MVBs in the Raji B cell remained unchanged ( Fig. 3a, and Supplementary Fig. S3 ). Similar results were obtained in experiments in which CH7C17 T cells, bearing an influenza hemagglutinin (HA) peptide-specific TCR, were conjugated to HA peptide-pulsed Hom2 B cells, thus confirming that antigen-induced formation of an IS polarizes T-cell MVBs to the contact site ( Fig. 3b,c ). Live cell imaging of CD63-GFP-expressing J77 T cells encountering SEE-pulsed Raji B cells revealed that the MVBs of the T cells move to the IS during the first 10 min ( Fig. 3d, and Supplementary Movie 1 ). 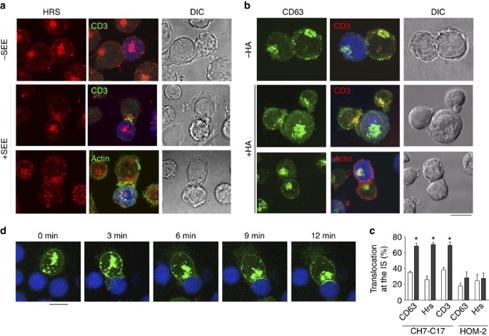Figure 3: MVBs in T cells translocate to the IS. (a) J77 T cells were conjugated with SEE-pulsed or non-pulsed Raji B cells loaded with CMAC (blue). After 30 min, cells were fixed and stained for the MVB marker Hrs (red), CD3 and actin (both green). Plates show maximal projections of confocal images and the DIC images. (b) CH7C17 T cells were conjugated with HA-loaded or non-loaded HOM2 B cells (blue). After 30 min, cells were fixed and stained for CD63 (green), CD3 and actin (both red). Plates show maximal projections of confocal images and the DIC images, scale bars applies toaandb. (c) Percentage of T and APC cells in which CD63, Hrs and CD3 relocalized to the T cell–APC contact area in the presence of HA peptide (filled bars) or its absence (open bars). Data are the arithmetic means±s.e.m. of four experiments. *P<0.03 compared with the absence of antigen (Mann–Whitney test). (d) Live cell imaging of J77-CD63-GFP cells seeded on fibronectin-coated coverslips and conjugated with SEE-primed Raji cells (blue). Cells were monitored by time-lapse confocal microscopy at 30 s intervals. Plates show maximal projections of confocal images. Scale bars, 10 ìm. Figure 3: MVBs in T cells translocate to the IS. ( a ) J77 T cells were conjugated with SEE-pulsed or non-pulsed Raji B cells loaded with CMAC (blue). After 30 min, cells were fixed and stained for the MVB marker Hrs (red), CD3 and actin (both green). Plates show maximal projections of confocal images and the DIC images. ( b ) CH7C17 T cells were conjugated with HA-loaded or non-loaded HOM2 B cells (blue). After 30 min, cells were fixed and stained for CD63 (green), CD3 and actin (both red). Plates show maximal projections of confocal images and the DIC images, scale bars applies to a and b . ( c ) Percentage of T and APC cells in which CD63, Hrs and CD3 relocalized to the T cell–APC contact area in the presence of HA peptide (filled bars) or its absence (open bars). Data are the arithmetic means±s.e.m. of four experiments. * P <0.03 compared with the absence of antigen (Mann–Whitney test). ( d ) Live cell imaging of J77-CD63-GFP cells seeded on fibronectin-coated coverslips and conjugated with SEE-primed Raji cells (blue). Cells were monitored by time-lapse confocal microscopy at 30 s intervals. Plates show maximal projections of confocal images. Scale bars, 10 ìm. Full size image The IS promotes the transfer of exosomes from the T cell to the APC To investigate whether the IS promotes the transfer of exosomes from T cells to APCs, CD63-GFP T cells were cultured with Raji cells (stained blue with chloromethyl derivative of aminocoumarin (CMAC)) for 16 h, by which most stage conjugates will have separated. The coculture was analysed by flow cytometry for the transfer of CD63-GFP. SEE-pulsed Raji cells acquired CD63-GFP from the T cells, whereas transfer in the absence of SEE was negligible ( Fig. 4a ). No transfer of GFP signal was detected when the assay was performed in the opposite direction (from Raji-CD63-GFP to J77 cells; Fig. 4a ) or when using J77 cells overexpressing non-exosomal membrane or cytoplasmic proteins (CD69-GFP and GFP; Fig. 4b ). In addition, we also detected transfer of other molecules related to exosomes and vesicles, such as CD38 (ref. 31 ) and LAT ( Supplementary Fig. S4 ). 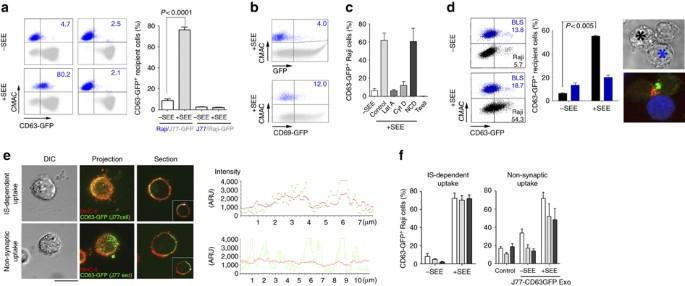Figure 4: Ag recognition induces transfer of exosomes from T cell to APC. (a) Left: J77-CD63-GFP donor cells were conjugated with SEE-primed or unprimed Raji cells (recipient, in blue). Right: Raji-CD63-GFP donor cells (±SEE) were conjugated with blue-labeled J77 recipients. After 16 h, cocultures were analysed by flow cytometry. Bar chart shows the percentage±s.e.m. of positive recipient cells (n=9,P<0.001, Student'st-test). (b) J77 cells transfected with CD69-GFP or GFP were conjugated with SEE-primed Raji cells (blue) and analysed as ina. (c) FACS analysis of the percentage of GFP-positive Raji cells after incubation with J77-CD63-GFP cells in contact with coculture as ina(control), in the presence of inhibitors of actin (latrunculin-A, LatA or cytochalasin-D, CytD) or tubulin (nocodazol, NCD), or after incubation with separation of donors and recipients by a 0.4 μm pore-size transwell membrane (Twell). T cells in transwells were activated with CD3+CD28 Abs and Raji cells were loaded with SEE. (d) J77-CD63-GFP donor cells were conjugated with a 1:1 mix of two B cell lines: Raji cells (black) and BLS-1 cells (blue) and analysed as ina. Bar chart shows percentages±s.e.m. of positive recipient cells (n=6,P<0.005, Mann–Whitney test). Maximal projections of confocal images and the DIC of a triple conjugated formed by J77-CD63-GFP (green), Raji cells (black asterisk) and BLS-1 (CMAC stained and blue asterisk), stained for CD3 (red) are shown, scale bar shown ine. (e) Confocal analysis of Raji cells that acquired CD63-GFP directly from J77-CD63-GFP after IS formation (IS-dependent transfer) or after external administration of CD63-GFP exosomes isolated from J77-CD63GFP supernatants (non-synaptic uptake). Cells were stained for MHC-II (red). Images show maximal projections of confocal images, one representative confocal section, and the DIC images. Plots show cell perimeter fluorescence intensity profiles of the green and the red signals. ARU: arbitrary relative units. Scale bar, 10 ìm. (f) Raji cells (±SEE) were treated as ine. FACS analysis of the effect of trypsin on the CD63-GFP content of Raji cells that acquired exosomes by IS-dependent transfer or non-synaptic uptake. White bars, control; grey bars, 10 min trypsin; black bars, 10 min+10 min trypsin. Bar chart shows percentages±s.e.m. of positive cells (n=3). Figure 4: Ag recognition induces transfer of exosomes from T cell to APC. ( a ) Left: J77-CD63-GFP donor cells were conjugated with SEE-primed or unprimed Raji cells (recipient, in blue). Right: Raji-CD63-GFP donor cells (±SEE) were conjugated with blue-labeled J77 recipients. After 16 h, cocultures were analysed by flow cytometry. Bar chart shows the percentage±s.e.m. of positive recipient cells ( n =9, P <0.001, Student's t -test). ( b ) J77 cells transfected with CD69-GFP or GFP were conjugated with SEE-primed Raji cells (blue) and analysed as in a . ( c ) FACS analysis of the percentage of GFP-positive Raji cells after incubation with J77-CD63-GFP cells in contact with coculture as in a (control), in the presence of inhibitors of actin (latrunculin-A, LatA or cytochalasin-D, CytD) or tubulin (nocodazol, NCD), or after incubation with separation of donors and recipients by a 0.4 μm pore-size transwell membrane (Twell). T cells in transwells were activated with CD3+CD28 Abs and Raji cells were loaded with SEE. ( d ) J77-CD63-GFP donor cells were conjugated with a 1:1 mix of two B cell lines: Raji cells (black) and BLS-1 cells (blue) and analysed as in a . Bar chart shows percentages±s.e.m. of positive recipient cells ( n =6, P <0.005, Mann–Whitney test). Maximal projections of confocal images and the DIC of a triple conjugated formed by J77-CD63-GFP (green), Raji cells (black asterisk) and BLS-1 (CMAC stained and blue asterisk), stained for CD3 (red) are shown, scale bar shown in e . ( e ) Confocal analysis of Raji cells that acquired CD63-GFP directly from J77-CD63-GFP after IS formation (IS-dependent transfer) or after external administration of CD63-GFP exosomes isolated from J77-CD63GFP supernatants (non-synaptic uptake). Cells were stained for MHC-II (red). Images show maximal projections of confocal images, one representative confocal section, and the DIC images. Plots show cell perimeter fluorescence intensity profiles of the green and the red signals. ARU: arbitrary relative units. Scale bar, 10 ìm. ( f ) Raji cells (±SEE) were treated as in e . FACS analysis of the effect of trypsin on the CD63-GFP content of Raji cells that acquired exosomes by IS-dependent transfer or non-synaptic uptake. White bars, control; grey bars, 10 min trypsin; black bars, 10 min+10 min trypsin. Bar chart shows percentages±s.e.m. of positive cells ( n =3). Full size image To define the requirement for cell–cell contact, we separated donor and recipient populations by a 0.4 μm pore-size Transwell membrane. J77-CD63-GFP T cells in transwell assays were treated with anti-CD3 plus anti-CD28 to activate them and therefore enhance exosome release [32] ( Supplementary Fig. S2b ). Although T cell CD69 levels indicated that cells had been activated to the same extent as after formation of an IS, no CD63-GFP was detected on APC recipient cells, whether or not these were loaded with SEE ( Fig. 4c and Supplementary Fig. S5a ). Also, in contact (non-Transwell) cocultures, stimulation with CD3 and CD28 Abs in the absence of SEE did not support CD63-GFP transfer ( Supplementary Fig. S5b,c ). Moreover, CD63-GFP transfer in standard (in the presence of SEE) contact cocultures was abolished by addition of the actin cytoskeleton inhibitors cytochalasin-D and latruculin-A, which disrupt the IS [33] , whereas the microtubule inhibitor nocodazol had no effect ( Fig. 4c ). These results indicate that cell–cell contact and T-cell activation by themselves do not support exosomal transfer. To confirm that the exosomal transfer requires a functional IS, we cocultured J77-CD63-GFP T cells with a mix of Raji B cells and BLS-1 B cells, which lack HLA class II and cannot form an IS [34] . After 16 h, GFP signal was detected on SEE-primed Raji B cells ( Fig. 4d ). In contrast, BLS-1 B cells did not trigger CD63 translocation ( Fig 4d , right panel) or CD3 clustering. These findings indicate that although T and APCs can both take up immune exosomes, cognate immune interactions promote the transfer of exosomes from the T lymphocyte to the APC and their unidirectional acquisition by the conjugated APC. We next analysed the mechanism of exosome uptake by APCs. In post-conjugated Raji cells, which had acquired CD63-GFP on IS formation, the CD63-GFP co-localized at the plasma membrane with endogenous major histocompatibility complex (MHC)-II molecules, indicating that the exosomes either remained attached or had fused with the cell surface. Intensity profiles around the cell perimeter indicate similar distributions of both molecules in the plasma membrane ( Fig. 4e ). In contrast, in Raji cells that had acquired CD63-GFP by direct addition of exosomes isolated from J77-CD63-GFP cells (non-synaptic uptake), the GFP signal appeared as aggregates attached to the plasma membrane and did not coincide with endogenous plasma membrane MHC-II ( Fig. 4e ). To find out whether T cell exosomes are fused or only adhered to the APC plasma membrane, we treated the Raji cells with trypsin. Trypsin treatment did not decrease the GFP signal acquired by SEE-loaded Raji cells from conjugated J77-CD63-GFP, indicating that exosomes transferred on immune synapsis can fuse with the APC plasma membrane or be internalized ( Fig. 4f ). In contrast, trypsin decreased the fluorescence signal of Raji cells that acquired CD63-GFP by non-synaptic uptake ( Fig. 4f ). These results suggest that the IS might not only promote the secretion of exosomes from T cell to APC, but might also induce the fusion of these exosomes with the plasma membrane of the recipient cell. The IS promotes the transfer of exosomal miRNA To demonstrate delivery of exosomal miRNA from T cell to APC after IS formation, we stably overexpressed miR-335 in J77-CD63-GFP T cells ( Fig. 5a ). This miRNA is not normally expressed in the donor (J77) or recipient (Raji) cells, but is sorted to the exosomes of primary immune cells (DCs and T lymphoblasts; Figs 1c and 5a , and Supplementary Data 1 ). J77-CD63-GFP cells expressing miR-335 (J-335) were cocultured with unprimed or SEE-primed Raji B cells (stained blue with CMAC), and after 24 h the Raji cells were sorted by flow cytometry ( Supplementary Fig. S6 ) and their miR-335 content analysed by reverse transcription PCR. miR-335 was transferred to Raji cells only in the presence of SEE ( Fig. 5b ). Raji cells that acquired high amounts of CD63-GFP contained correspondingly high amounts of miR-335, demonstrating correlation between the transfer of miR-335 and exosomal proteins ( Fig. 5b ). To demonstrate that miR-335 is not expressed de novo in Raji cells after IS formation, we repeated the experiment with J77-CD63-GFP cells stably overexpressing miR-101 (J-101); conjugation with these cells did not induce expression of miR-335 in Raji cells ( Fig. 5b ). The ability of a peptide antigen-specific IS to transfer miRNA was further demonstrated in HA-loaded CH7C17 cells overexpressing miR-335 (C-335) and conjugated to Hom-2 cells ( Fig. 5c ), demonstrating antigen-specific directional transfer of exosomal miRNA from T cell to APC. We also investigated the transfer of endogenous miRNAs by primary SEE-specific T lymphocytes. These cells transferred endogenous miR-335 and miR-92 to Raji APCs in a SEE-specific manner ( Fig. 5d ). 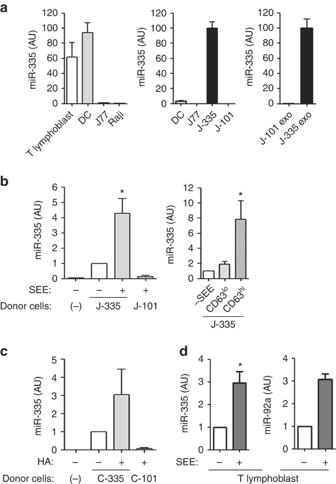Figure 5: Exosomal miRNA-335 is transferred from T cell to APC in an Ag-specific manner. (a) Levels of miR-335 were assessed by quantitative reverse transcription PCR (qRT–PCR) in primary dendritic cells and T lymphoblasts, and in Raji and J77 cells. J77-CD63-GFP cells were stably transduced with miR-335 (J-335 cells) or miR-101 (J-101 cells), and miR-335 levels were determined by qRT–PCR in cells and derived exosomes. Data are representative of three experiments (mean and s.e.m.) (b) miR-335 levels in SEE-primed Raji cells sorted 24 h after conjugation with J-335 cells. J-101 were used as control donor cells. Left panel, Data are representative of seven independent experiments (mean and s.e.m),P=0.014 (one-samplet-test). Right panel,n=5 independent experiments;P=0.04 (one-samplet-test); error bars represent s.e.m. (c) miR-335 levels in HA-primed HOM-2 cells sorted 24 h after conjugation with CH7C17 cells overexpressing miR-335 (C-335). CH7C17 cells overexpressing miR-101 (C-101) were used as control donor cells. Data are representative of five experiments (mean and s.e.m.). (d) miR-335 and miR-92a levels in SEE-primed Raji cells sorted 24 h after conjugation with primary T lymphoblasts-expressing miR-335 and miR-92a endogenously. Data are representative of three experiments (mean and s.e.m.), *P=0.026 (one-samplet-test) AU, arbitrary units. Figure 5: Exosomal miRNA-335 is transferred from T cell to APC in an Ag-specific manner. ( a ) Levels of miR-335 were assessed by quantitative reverse transcription PCR (qRT–PCR) in primary dendritic cells and T lymphoblasts, and in Raji and J77 cells. J77-CD63-GFP cells were stably transduced with miR-335 (J-335 cells) or miR-101 (J-101 cells), and miR-335 levels were determined by qRT–PCR in cells and derived exosomes. Data are representative of three experiments (mean and s.e.m.) ( b ) miR-335 levels in SEE-primed Raji cells sorted 24 h after conjugation with J-335 cells. J-101 were used as control donor cells. Left panel, Data are representative of seven independent experiments (mean and s.e.m), P =0.014 (one-sample t -test). Right panel, n =5 independent experiments; P =0.04 (one-sample t -test); error bars represent s.e.m. ( c ) miR-335 levels in HA-primed HOM-2 cells sorted 24 h after conjugation with CH7C17 cells overexpressing miR-335 (C-335). CH7C17 cells overexpressing miR-101 (C-101) were used as control donor cells. Data are representative of five experiments (mean and s.e.m.). ( d ) miR-335 and miR-92a levels in SEE-primed Raji cells sorted 24 h after conjugation with primary T lymphoblasts-expressing miR-335 and miR-92a endogenously. Data are representative of three experiments (mean and s.e.m. ), * P =0.026 (one-sample t -test) AU, arbitrary units. Full size image To confirm that miRNA transfer is mediated by exosomes, we blocked exosome production in J-335 cells. Ceramide, biosynthesis of which is regulated by neutral sphingomyelinase-2 (nSMase2), triggers the budding of exosomes into MVBs, and inhibition of nSMase2 therefore reduces the secretion of CD63-containing exosomes [35] and miRNAs [36] . Accordingly, the secretion of exosomes by J77 cells was impaired when nSMase2 activity was reduced either by addition of the inhibitor manumycin-A ( Fig. 6a ) or by small hairpin RNA (shRNA) silencing ( Fig. 6b and Supplementary Fig. S7a ). Targeting of nSMase2 activity inhibited the IS-dependent transfer of CD63-GFP ( Fig. 6c,d ) and miRNA-335 ( Fig. 6e,f ). Transfer of CD63-GFP and miR-335 was also blocked by brefeldin ( Fig. 6c,e ), which inhibits the guanine nucleotide-exchange protein BIG2 and regulates the constitutive release of exosome-like vesicles [37] . Exosome secretion and CD63-GFP transfer by J-335 cells was also inhibited by shRNA silencing of the Rab GTPase Rab27a, which is implicated in the exosomal release pathway [38] ( Supplementary Fig. S7b–d ). In contrast, transfer of CD63-GFP occurred normally from Hrs-interfered J77 T cells ( Supplementary Fig. S7e and Fig. 6d ), in agreement with previous studies that demonstrated that the ESCRT system is unnecessary for the release of exosomes and miRNA [35] , [36] . 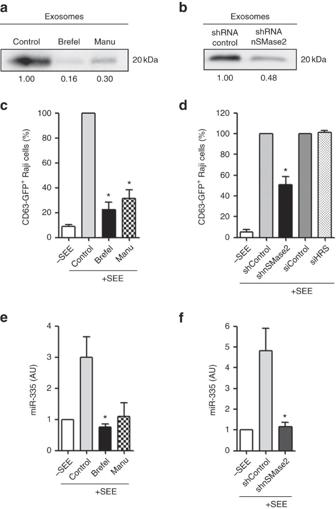Figure 6: Inhibition of exosome biogenesis impairs transfer of exosomal miRNAs and proteins through the IS. (a) J77 cells were cultured in exosome-depleted medium for 24 h, in the presence of inhibitors of nSMase2 (manumycin-A, Manu) or BIG2 (brefeldin, Brefel). Purified exosomes secreted by equal numbers of control or treated cells were analysed by immunoblotting for the presence of the exosome marker CD81. Densitometric analyses were performed, and the ratio between the treated and the control condition is shown. (b) CD81 immunoblot of exosomes purified from equal numbers of cells transduced with control or nSMase2 shRNA. Densitometric analyses were performed, and the ratio between the silenced and the control condition is shown. (c) FACS analysis of the CD63-GFP content of Raji recipients cells after conjugation with J-335 cells in the presence of manumycin or brefeldin. Data are the percentage±s.e.m. of Raji-GFP-positive recipient cells relative to the SEE-loaded control condition.n=5 independent experiments;P≤0.001 (one-samplet-test). (d) FACS analysis of the CD63-GFP content of Raji recipient cells after coculture with J77-CD63GFP cells expressing shnSMase2 or siHrs. Data are the percentage±s.e.m. of Raji-GFP-positive recipient cells relative to the SEE-loaded control condition.n=8 independent experiments, *P=0.0005 (one-samplet-test). (e) Quantitative reverse transcription PCR (qRT–PCR) analysis of miR-335 in Raji cells sorted after conjugation with J-335 cells in the presence of manumycin or brefeldin.n=3 independent experiments; *P=0.03 (unpairedt-test). (f) qRT–PCR analysis of miR-335 in Raji cells sorted after conjugation with J-335 transduced with shnSMase 2 or shControl.n=4 independent experiments; *P=0.012 (unpairedt-test); error bars represent s.e.m. Figure 6: Inhibition of exosome biogenesis impairs transfer of exosomal miRNAs and proteins through the IS. ( a ) J77 cells were cultured in exosome-depleted medium for 24 h, in the presence of inhibitors of nSMase2 (manumycin-A, Manu) or BIG2 (brefeldin, Brefel). Purified exosomes secreted by equal numbers of control or treated cells were analysed by immunoblotting for the presence of the exosome marker CD81. Densitometric analyses were performed, and the ratio between the treated and the control condition is shown. ( b ) CD81 immunoblot of exosomes purified from equal numbers of cells transduced with control or nSMase2 shRNA. Densitometric analyses were performed, and the ratio between the silenced and the control condition is shown. ( c ) FACS analysis of the CD63-GFP content of Raji recipients cells after conjugation with J-335 cells in the presence of manumycin or brefeldin. Data are the percentage±s.e.m. of Raji-GFP-positive recipient cells relative to the SEE-loaded control condition. n =5 independent experiments; P ≤0.001 (one-sample t -test). ( d ) FACS analysis of the CD63-GFP content of Raji recipient cells after coculture with J77-CD63GFP cells expressing shnSMase2 or siHrs. Data are the percentage±s.e.m. of Raji-GFP-positive recipient cells relative to the SEE-loaded control condition. n =8 independent experiments, * P =0.0005 (one-sample t -test). ( e ) Quantitative reverse transcription PCR (qRT–PCR) analysis of miR-335 in Raji cells sorted after conjugation with J-335 cells in the presence of manumycin or brefeldin. n =3 independent experiments; * P =0.03 (unpaired t -test). ( f ) qRT–PCR analysis of miR-335 in Raji cells sorted after conjugation with J-335 transduced with shnSMase 2 or shControl. n =4 independent experiments; * P =0.012 (unpaired t -test); error bars represent s.e.m. Full size image Transferred miRNAs regulate gene expression on the APC To determine whether synaptically transferred miRNA-335 is functional in the recipient APC, we carried out luciferase reporter assays with full-length 3′-UTR constructs of the miR-335 target SOX4 and the miR-335-insensitive UBE2F [39] . Raji cells transfected with luciferase constructs were cocultured with J-335 cells and luciferase activity was assessed. Expression from the SOX4 3′-UTR was significantly reduced in SEE-primed Raji cells that had been in contact with J-335 cells, whereas expression from the UBE2F 3′-UTR was unaffected ( Fig. 7a ). Expression from these 3′-UTR reporters was not affected by coculture of Raji cells with J-101 cells, indicating that the process is not a general effect of IS formation, but rather involves the direct transfer of the specific miRNA. Reduction in luciferase activity after conjugate formation was also detected in Raji cells expressing base pairs 449–509 of the SOX4 3′-UTR, which encompasses the miR-335 seed sequence; and inhibition of luciferase expression was abolished by mutation of this sequence ( Fig. 7b ). The IS thus guides the transfer of functional miRNA from the T cell to the APC. Contrasting with IS-dependent miRNA transfer, addition of exosomes isolated from J-335 cells to transfected Raji cells had no effect on luciferase activity ( Fig. 7a,b ), indicating that any miR-335 acquired in this way was non-functional. 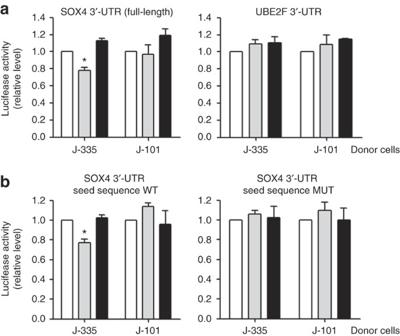Figure 7: Synaptically transferred miR-335 downregulates target gene expression in the APC. (a) Raji cells were transfected with reporter constructs consisting of the luciferase sequence placed upstream of the full-length 3′-UTR of either the miR-335-target gene SOX4 or the control gene UBE2F. Luciferase activity was assayed 24 h after coculture of SEE-loaded Raji with J77-miR-335 cells or control J-101 cells (synaptic transfer) or after addition of derived exosomes to SEE-loaded Raji cells (non-synaptic uptake). (b) Experiments as inaperformed with Raji recipient cells expressing the wild-type of mutated seed sequence for miR-335 from the SOX4 3′-UTR. Luciferase activities are shown relative to control incubations with untreated Raji cells. Data are means±s.e.m.;n=5 independent experiments, *P<0.05 (Newman–Keuls multiple comparison test). White bars, control; grey bars, synaptic transfer; black bars, non-synaptic transfer. Figure 7: Synaptically transferred miR-335 downregulates target gene expression in the APC. ( a ) Raji cells were transfected with reporter constructs consisting of the luciferase sequence placed upstream of the full-length 3′-UTR of either the miR-335-target gene SOX4 or the control gene UBE2F. Luciferase activity was assayed 24 h after coculture of SEE-loaded Raji with J77-miR-335 cells or control J-101 cells (synaptic transfer) or after addition of derived exosomes to SEE-loaded Raji cells (non-synaptic uptake). ( b ) Experiments as in a performed with Raji recipient cells expressing the wild-type of mutated seed sequence for miR-335 from the SOX4 3′-UTR. Luciferase activities are shown relative to control incubations with untreated Raji cells. Data are means±s.e.m. ; n =5 independent experiments, * P <0.05 (Newman–Keuls multiple comparison test). White bars, control; grey bars, synaptic transfer; black bars, non-synaptic transfer. Full size image The data presented here establish a highly efficient intercellular mechanism for the transfer of regulatory genetic information exclusively in the microenvironment of the IS. Unlike other examples of RNA transfer via microvesicles, where non-synaptic release potentially allows the exchange of genetic material at a distance, our data indicate that during cognate immune interactions there is a unidirectional transfer of miRNA from the T to the APC. This genetic communication is antigen driven and appears to be linked to the formation of the IS. The importance of exosome release in this process is demonstrated by the correlation of miRNA transfer with that of CD63 and by its blockade with inhibitors of exosome production. Cells release different types of vesicles into the extracellular space. Two types of vesicles can be distinguished depending on their cellular origin. Shedding vesicles are generated by budding from the plasma membrane into the extracellular space [40] , [41] , whereas exosomes have an endosomal origin in MVBs: MVBs either fuse with lysosomes for degradation or with the plasma membrane to release their intraluminal vesicles (ILVs) as exosomes. Mixed populations, containing shedding vesicles and exosomes, are referred as microvesicles. Microvesicles are increasingly recognized as important mediators of cell-to-cell communication [11] . They can transfer receptors, proteins, mRNA and miRNA to target cells via interaction with specific receptors. Microvesicles derived from embryonic stem cells have been reported to reprogramme haematopoietic progenitors through the delivery of mRNA [16] . The transfer of RNA species via microvesicles to endothelial cells induces angiogenesis [14] , [15] and progenitor mobilization [17] . In the immune system, exosomal transfer of mRNA occurs between mast cells [13] , and viral miRNAs secreted by EBV-infected cells can be taken up by uninfected recipient cells [18] . Synthetic miRNA mimetics and viral miRNAs have been reported to be transferred between leukocytes, although the direct involvement of exosomes/microvesicles in this case was not demonstrated [42] . Exchange of proteins between immune cells has been extensively reported, but the mechanism of this transfer remains unclear [43] . This phenomenon, which has been called trogocytosis, is considered to be an antigen-specific event that requires the formation of an IS. Our data suggest that the mechanism for the transfer of certain proteins during immune synapsis is the directional release of exosomes. In accordance with other reports, our data show that exosomes can be transferred between cells at a distance. However, in the case of immune cells, the presence of specific antigen induces the formation of an IS, and enhances this exosomal transition. ISs are highly organized cell–cell contacts where, on antigen recognition, T-cell activation is initiated and tuned. The generation of an IS involves the polarization of several T-cell organelles towards the APC. Among them, the MTOC, the Golgi apparatus and cytotoxic granules are required for effector functions, such as exocytosis of lytic granules by cytotoxic T cells or polarized secretion of cytokines by helper T cells [6] . However, not all cytokines are released directly at the IS; some, such as tumour necrosis factor or interleukin (IL)-4, are delivered via a multidirectional pathway [5] , [44] . The formation of an IS induces the polarization of T-cell MVBs towards the IS and enhances the discharge of exosomes (see ref. 32 and the present report). This localization suggests that the fusion of MVBs with the plasma membrane for exosome release might occur at the IS zone. Moreover, when CD63-GFP T cells were cocultured simultaneously with two B cell lines, only B cells presenting SEE were able to uptake the CD63-GFP signal, strongly indicating polarized, IS-dependent transfer. Further experimentation will be needed, however, to unequivocally determine whether exosomal transport occurs in a polarized manner through the IS or is multidirectional. Interestingly, CD63 was not transferred in T–B contact cocultures in the presence of stimuli that activate T cells without forming an IS. These results indicate that cell–cell contact and T-cell activation are not sufficient for the observed exosomal transfer, and that the formation of an IS is critical. For example, antigen might act on the recipient B cell to facilitate exosome uptake. Moreover, only exosomes acquired on IS formation appear to be functional in the recipient cell. These data suggest that, in addition to exchange of exosomes at a distance, the formation of an IS enhances this transfer and promotes the directional and functional release of T-cell exosomes to the APC. Complex mechanisms underlie the sorting of cargo into different populations of ILVs. Ubiquitinated proteins require the action of the ESCRT machinery to mediate degradative protein sorting [45] , whereas other cargos such as CD63 are sorted in a ceramide-dependent pathway that generates another population of ILVs destined for secretion as exosomes [35] . Our data and previous reports [18] , [46] indicate that not all miRNAs can be incorporated into exosomes, and therefore that the packaging of specific miRNA populations into exosomes is selective. However, the mechanisms controlling this sorting remain unclear. miRNAs incorporate into exosomes and are released via a ceramide-dependent pathway independent of the ESCRT machinery [36] . Moreover, as proteins of the RNA-induced silencing complex have been detected in exosomes [47] , it is feasible that association with RNA-induced silencing complex components controls the packaging of miRNAs in exosomes. Blocking MVB formation by ESCRT depletion results in impaired miRNA silencing [47] , [48] , thus suggesting that MVBs could be a miRNA crossroad to secretory pathway and gene silencing. Other potential mechanisms for the packaging of specific miRNAs in exosomes are 3′ modification and their association with target mRNA. Our mechanistic studies with chemical inhibitors and nSMase2 siRNA show that exosomal miRNAs are exchanged during IS formation via a ceramide-dependent, ESCRT-independent pathway. In accordance with previous reports, we observed that knocking down members of the Rab GTPases family inhibits exosome secretion [38] and the transfer of exosomal content during immune synapsis, whereas Hrs silencing has no effect. Our results show that the transfer of CD63 correlates with the transfer of one miRNA, miR-335, from the T cell to the APC. miRNA-335 is especially suitable for our technical approach, as it is expressed in primary leukocytes, is highly enriched in exosomes, and its expression is negligible in Raji B cells. It is feasible that other exosomal miRNAs can also be transferred during immune synapsis. Our data show that levels of miR-92a, another miRNA abundant in exosomes, increase in Raji cells after conjugation with T lymphoblasts. However, as this miRNA is endogenously expressed by B cells, we cannot distinguish between endogenous upregulation and horizontal transfer. Today there is no doubt that miRNAs are important modulators of the immune system [21] , [22] , [49] . Modification of gene expression in recipient cells by transferred genetic material could account for several exosome functions. This exosomal transfer of regulatory RNAs is potentially a powerful means of orchestrating gene expression during the generation of the immune response, and increases the complexity of communication between cells. Our data demonstrate that miRNAs transferred during immune synapsis can be functional in the recipient cell, and suggest that T cell-derived miRNAs regulate specific targets in APCs. As an example, we demonstrate that miRNA-335 downregulates translation of SOX-4 mRNA. This miRNA-335 target gene has recently been reported in breast cancer cells [39] . In contrast, Raji cells that were exposed to isolated exosomes without cellular contact showed no miRNA activity, and the exosomal protein signal could be removed by trypsin treatment. How exosomes deliver their content to recipient cells remains unclear. It has been proposed that, depending on the origin of exosomes and the identity of the recipient cells, exosomes might be internalized by endocytosis [50] , phagocytosis [51] , [52] or by direct fusion with the plasma membrane [53] . Whatever the mechanism, the differences we observed between IS-dependent exosomal transfer and uptake without cell contact support the notion that the immune synapse promotes the transfer of miRNA-loaded exosomes by T cell and facilitates functional delivery of the miRNA into the APC. Cells and reagents The human Jurkat-derived T-cell lines J77cl20 (TCR Vαl. 2 Vβ8) [54] and CH7C17 (Vβ3 TCR specific for HA peptide) [55] and the lymphoblastoid B-cell lines Raji (Burkitt lymphoma), HOM-2 (HLA-DR1 EBV-transformed) and BLS-1 (HLA class II-null B-LCL, generated from cells of patients with type II Bare lymphocyte syndrome) [34] were cultured in RPMI (Sigma) containing 10% fetal bovine serum (Invitrogen). Stable cell line clones overexpressing CD63-GFP were generated by transfection and selection with G418 (1 mg ml −1 ). The CD63-GFP cell lines were subsequently transduced by lentiviral infection to overexpress miR-335 or miR-101 and selected with blasticidin (5 μg ml −1 ) and G418 (2 mg ml −1 ); the resulting cell lines were designated as follows: J77-CD63-GFP-miR335 (J-335), J77-CD63-GFP-miR101 (J-101), CH7C17-CD63-GFP-miR335 (C-335) and CH7C17-CD63-GFP-miR101 (C-101). Human peripheral blood mononuclear cells were isolated from buffy coats from healthy donors by separation on a biocoll gradient (Biochrom). After 30 min of adhesion step at 37 °C, non-adherent cells were cultured 2 days in the presence of phytohemagglutinin (5 μg ml −1 ) to induce lymphocyte proliferation. To obtain T lymphoblasts, IL-2 (50 U ml −1 ) was added to the medium every 2 days for a time period of 8 days. To obtain SEE-specific T lymphoblasts, cells were cultured 10 days in the presence of SEE. After adhesion step, adherent monocytes were cultured in the presence of IL-4 and granulocyte macrophage colony-stimulating factor to induce their differentiation into DCs. Maturation of DCs was promoted by adding lipopolysaccharide [56] . The fluorescent cell trackers CMAC and BCECF (bis-carboxyethyl-carboxyfluorescein) were from Molecular Probes. Latrunculin-A (LatA), manumycin-A, nocodazol (NCD), cytochalasin-D (CytD) and recombinant human fibronectin and poly- L -lysine were from Sigma. The following anti-human antibodies were produced in the laboratory: anti-CD63 mAb (Tea 3/18), anti-CD3 mAb (t3b), anti-CD45 (D3/9) and anti-MHC-II (DCIS1/21). Phycoerythrin-anti-human CD63 was from BD Biosciences, anti-mouse CD63 mAb (NKI/C-3) and anti-Hrs were from HGS Abcam, and anti-CD81 mAb (5A6) from Santa Cruz. Lentiviruses-expressing shRNA were obtained from the Open Biosystems Expression Arrest RNAi consortium (TRC) library. Clone ID of the shRNA used were: TRCN0000005294 for RAB27A, and TRCN0000048947, TRCN0000048946, TRCN0000048945, TRCN0000048944, TRCN0000048943 for nSMAse2 (SMPD3). Hrs was knocked down with a pair of RNA sequences (5′-CGACAAGAACCCACACGUCtt-3′, together with 5′-AAGCGGAGGGAAAGGCCACUUTT-3′) from Ambion. Control sequences were On-Target plus non-targeting siRNA no. 1 and 2 (Dharmacon) and the sequence 5′-UUCUCCGAACGUGUCACGUtt-3′. Cell transfection J77 or Raji cells were transfected with CD63-GFP, CD44-GFP, EGFP, LAT-GFP or CD38-GFP plasmids by electroporation [57] . Cells were resuspended in Opti-MEM (GIBCO; 5×10 7 cells per ml) with 20 μg of DNA plasmid and electroporated with Gene Pulser Xcell (Bio-Rad) at 1200 μFa, 240 mV during 30 ms at 4 mm Bio-Rad cuvettes (Bio-Rad). CD63-GFP-positive cells were FACS sorted, cloned and cultured in RPMI containing 2 mg ml −1 G418 (Invitrogen). Lentiviral infection J77-CD63-GFP cells overexpressing miRNA-355 or miRNA-101 were generated by lentiviral infection. HEK293T cells were co-transfected (Lipofectamine2000; Invitrogen) with miRVec plasmids encoding the desired miRNA (Geneservice) and pCL-Ampho plasmid (RetroMax). Supernatants were collected after 48–72 h, filtered (0.45 μm) and added to J77-CD63-GFP cells. Cells were centrifuged (1,200 g , 2 h) and incubated for 4 h at 37 °C. Medium was replaced with RPMI-containing blasticidin (5 μg ml −1 ) and G418 (2 mg ml −1 ). To silence RAB27A and nSMase2, HEK293T cells were co-transfected with corresponding shRNA pLKO system plasmids (Open Biosystems) and pCMV-ΔR8.91-(Delta 8.9) and pMD2.G-VSV-G. Supernatants were added to J77-CD63-GFP-miR-335 (J-335) cells, which were cultured in RPMI containing 4 μg ml −1 puromcyin. Exosome purification Donor cells were cultured in RPMI-1640 supplemented with 10% FBS (depleted of bovine exosomes by overnight centrifugation at 100,000 g ), and exosomes were prepared from cell supernatants by several centrifugation and filtration steps [29] . Briefly, cells were centrifuged (320 g for 5 min) and the supernatant filtered through 0.22 μm membranes. Exosomes were pelleted by ultracentrifugation at 100,000 g for 60 min at 4 °C (Beckman Coulter Optima L-100 XP, Beckman Coulter). RNA isolation Total RNA was extracted with TRIzol reagent (Invitrogen) and the miRNeasy mini kit (Quiagen), and was screened for purity and concentration in a Nanodrop-1000 Spectrophotometer (Thermo Scientific). RNA integrity was assessed by ethidium bromide labelling on a 1.5% agarose gel. MicroRNA analysis The Agilent 2100 Bioanalyzer (Agilent) for total RNA (RNA nano chips) and for small RNA (small RNA chips) were used to assess the large and small RNA profiles in cells and exosomes. Microarray experiments were performed using the human microRNA microarray from Agilent. Arrays were performed on three different RNA preparations from Raji and J77 cells and their exosomes, and two preparations each from human DCs and their exosomes. Quantitative real-time-PCR Mature miRNA and mRNA quantification was performed by TaqMan real-time PCR (Applied Biosystems) according to the manufacturer's instructions. The following TaqMan miRNA Assays and TaqMan Gene expression Assays (Applied Biosystems) were used: hsa-miR-335 (000546), hsa-miR-92a (000431), RAB27A (Hs00608302_m1) and SMPD3 (nSMase2) (Hs00218713_m1). HY3 (001214) and RNU19 (001003) were used as endogenous controls for miRNA, whereas GAPDH (Hs02758991_g1) and HPRT (Hs01003267_m1) were used as endogenous controls for mRNA (all from Applied Biosystems). Reactions were performed in triplicate in 10 μl volumes. Quantitative miRNA or mRNA expression data were acquired and analysed using the ABI Prism 7900HT Sequence Detection System (Applied Biosystems). Data were further analysed using Biogazelle QBasePlus software (Biogazelle), and results are expressed in arbitrary units. Non-synaptic uptake experiments Exosomes were purified as described above and added to recipient cells in a ratio 1:25 (recipient:donor cells). After 16 h, recipient cells were analysed by flow cytometry. Conjugate formation To distinguish B cells from T cells, B cells (Raji or Hom2) were loaded with the blue fluorescent tracker CMAC [58] . B cells were incubated with SEE (Toxin Technology) or HA peptide (New England Peptide) as appropriate, and mixed with J77 cells (native or expressing CD63-GFP±miR-335 or miR-101) or CH7C17 cells at a ratio of 1:8. Conjugation at 37 °C was continued for times indicated in each case. Where indicated, J77 cells were preincubated with manumycin-A (10 μM), brefeldin (10 mg ml −1 ), nocodazol (5 μM), cytochalasin-D (20 μM) or latrunculin-A (1 μM). In experiments with Raji-CD63-GFP cells, J77 cells were labelled with CMAC. Where indicated, Raji and J77 cells were prevented from coming into direct contact by separating with a 0.4 μm pore-size transwell membrane (Costar). This allows the passage of exosomes but precludes direct cell–cell interaction. When indicated, T cells were activated with phorbol myristate acetate (50 ng ml −1 ) plus Ionomycin (0.5 μg ml −1 ), anti-CD3 plus anti-CD28 (both at 5 μg ml −1 ) or SEE (0.5 μg ml −1 ). Fluorescence confocal microscopy For immunofluorescence assays, cells were plated onto slides coated with poly- L -lysine (50 μg ml −1 ), incubated for 30 min, fixed, blocked and stained with the indicated primary antibodies (5 μg ml −1 ) followed by alexa488- or Rhodamine Red X-labeled secondary antibodies (5 μg ml −1 ). For live-cell imaging, Raji (preloaded with CMAC and SEE) and J77-CD63-GFP cells were added to coverslips coated with fibronectin (20 μg ml −1 , Sigma), mounted in Attofluor open chambers (Molecular Probes), and maintained at 37 °C in a 5% CO 2 atmosphere. Samples were examined with a Leica SP5 confocal microscope (Leica) fitted with a ×63 objective, and images were processed and assembled using Leica software. Flow cytometry analysis and sorting Cell samples were analysed with a FACSCanto flow cytometer and FACSDiva software (BD Biosciences). Viable cells were identified by propidium iodide exclusion. Singlet cells were discerned with a stringent multiparametric gating strategy based on FSC and SSC (pulse width and height). T cells and APCs were distinguished by CMAC staining and GFP fluorescence. Cells were sorted on a FACSAria flow cytometer (BD Biosciences). Raji cells were isolated after coculture with T cells by sorting for CMAC-positive singlet cells. Where indicated, Raji cells were also sorted based on CD63-GFP levels. Immunoblotting Cells or exosomes were lysed in RIPA (1% NP40, 0.5% deoxycholate, 0.1% SDS in TBS), with a cocktail of protease inhibitors (Complete, Roche). Proteins were separated in 10% acrylamide/bisacrylamide gel and transferred to a nitrocellulose membrane. Proteins were visualized with LAS-3000 after membrane incubation with specific antibodies (5 μg ml −1 ) and secondary antibodies conjugated to peroxidase (5 μg ml −1 ). Band intensities were quantified using WCIF Image J software and results are expressed relative to the control condition. UTR reporter assays Psicheck2 dual luciferase reporter vectors (Promega) cloned with the full-length 3′-UTRs of SOX4 and UBE2F and the SOX4 3′-UTR segment (base pairs 449–509) containing the wild-type or mutated (base pair 483) miR-335 seed sequence were a gift from Dr Massagué [39] (Memorial Sloan-Kettering Cancer Center, New York). Raji cells were transfected by electroporation and, 16 h later, cocultured with J-335 or J-101. After 24 h, cells were lysed and the ratio of Renilla and Firefly luciferase activities was measured by the dual luciferase assay (Promega). Statistical analysis Microarray data were normalized by the variance stabilization normalization (VSN) method [59] , and statistics were analysed with linear models as implemented in the limma Bioconductor package [60] . For statistical analysis of other experiments, data were analysed by unpaired t -test or one-sample t -test as stated in each case and the P -value was calculated. Accession codes: The microarray data have been deposited in NCBI's Gene Expression Omnibus and are accessible through GEO Series accession number GSE27997 . How to cite this article: Mittelbrunn, M. et al . Unidirectional transfer of microRNA-loaded exosomes from T cells to antigen-presenting cells. Nat. Commun. 2:282 doi: 10.1038/ncomms1285 (2011).